Forward models of repetition suppression depend critically on assumptions of noise and granularity 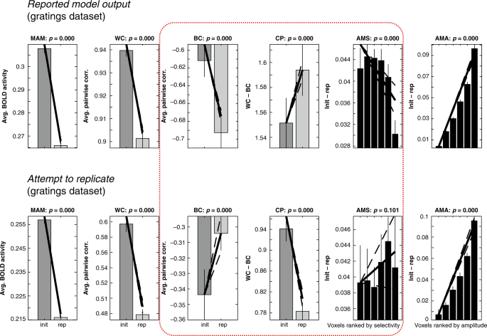Fig. 1: Noise parameters influence feed-forward models of fMRI-pattern correlations. Top row: pattern of results reported by Alink et al. for the winning parameter combination [a= 0.8,b= 0.4,σ= 0.4] for the grating dataset (cf. Supplementary Fig.4in Alink et al.). The direction (increase or decrease when comparing initial and repeated responses) of the six empirically observed data-features (cf. Figure 3 in Alink et al.) is only observed when uniformly distributed noise in the interval [0, 0.1] is added to the simulated brain patterns. Bottom row: the qualitative pattern of results observed for the winning parameter combination shown in the top row changed substantially when adding zero-mean Gaussian noise with a standard deviation of 0.1 instead of uniformly distributed noise. Of particular interest, the data-features BC, CP, and AMS are (shown within a red box) no longer qualitatively consistent with the empirical observations. Compare the corresponding slopes of lines in the top and bottom rows. Init initial presentation, rep repeated presentation, MAM mean amplitude modulation, WC within-class correlation, BC between-class correlation, CP “classification performance” (CP = WC − BC), AMS amplitude modulation by selectivity, AMA amplitude modulation by amplitude. Solid bars indicate mean of each condition and error bars 95% confidence intervals given the (simulated) between-participant variability. Diagonal lines indicate the slope of linear contrasts across conditions, and dashed lines indicate 95% confidence interval of the slope. See Alink et al. for methodological details and proposed interpretation of error bars andpvalues above each subpanel. In our view, given that arbitrary modeling choices determine the across-subject variability produced by the model, the reported error bars and accompanyingpvalues have therefore little, if any, statistical meaning. 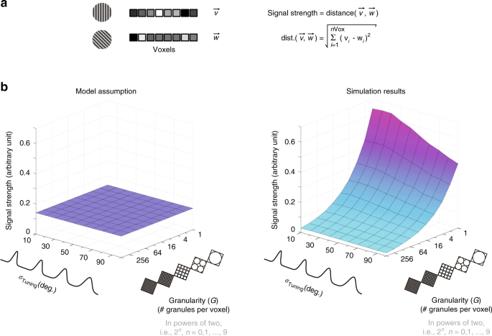Fig. 2: Noise amplitude and signal strength influence empirically observed fMRI–pattern correlations. afMRI patterns formed by concatenating responses across voxels for each of two experimental conditions—here, visual gratings oriented either 45° or 90° from the horizontal. The strength of the signal component distinguishing the brain responses associated with these two gratings can be quantified as the Euclidean distance between these two spatially distributed brain response patterns, treated as vectors, and denoted here as\(\vec v\)and\(\vec w\).bSimulation results: signal strength as a function of tuning bandwidth and granularity. In the class of models implemented by Alink et al., the tuning bandwidth of feature-tuned neural populations has been parametrized by Gaussian distributions. The preferred orientation of each neural population is described byμTuning, whileσTuningdescribes how tightly tuned each population is about its preferred orientation. In turn, the level of granularity of simulated fMRI data has been controlled by a positive integer (G) specifying the number of similarly tuned neural clusters, here referred to as granules, assumed to be sampled by each voxel13. The 3D surface shown to the right under the label “Simulation results” clearly demonstrates that granularity (x-axis), as well as tuning width (y-axis), influence the strength of simulated fMRI patterns. For each admissible parameter combination ofGandσTuningthez-axis indicates the average strength (across 25 randomly seeded simulations) of the signal distinguishing the fMRI response patterns denoted by\(\vec v\)and\(\vec w\). The full range of simulated granularity levels is [1, 512] (2n, withn= 0, 1, …, 9 granules per voxel). A dramatic effect of granularity on signal strength can be noted along thex-axis. If granularity were irrelevant, the observed monotonically decreasing curve would be instead a flat line. Given that pairwise correlations are known to be determined by noise amplitude as well as signal strength, this simulation demonstrates that the validity of inferences regarding neural coding based on fMRI–pattern correlations depend on granularity assumptions as well as noise parameters. Further information on research design is available in the Nature Research Reporting Summary linked to this article.